Sodium and potassium competition in potassium-selective and non-selective channels Potassium channels selectively conduct K + , primarily to the exclusion of Na + , despite the fact that both ions can bind within the selectivity filter. Here we perform crystallographic titration and single-channel electrophysiology to examine the competition of Na + and K + binding within the filter of two NaK channel mutants; one is the potassium-selective NaK2K mutant and the other is the non-selective NaK2CNG, a CNG channel pore mimic. With high-resolution structures of these engineered NaK channel constructs, we explicitly describe the changes in K + occupancy within the filter upon Na + competition by anomalous diffraction. Our results demonstrate that the non-selective NaK2CNG still retains a K + -selective site at equilibrium, whereas the NaK2K channel filter maintains two high-affinity K + sites. A double-barrier mechanism is proposed to explain K + channel selectivity at low K + concentrations. Potassium channels are tetrameric cation channels defined by their selective and efficient conduction of potassium ions across the lipid membrane to the exclusion of other ions, most notably sodium [1] . This discrimination is remarkable given the sub-angstrom difference in radius between sodium and potassium, and the fact that K + channels can pass ions at up to diffusion-limited rates. This selection occurs within part of the ion channel pore known as the selectivity filter, which is formed by the conserved signature sequence TVGYGD [2] , [3] . The filter of a channel tetramer assembles into a unique structure with four in-line potassium-binding sites, where the conducting ions are directly coordinated by carbonyls of the peptide backbone or the hydroxyl of the threonine side chain [4] . Although the sequence and structure responsible for mediating selectivity have been known for some time, the means by which selectivity is achieved remains under continued debate. Although initial structural studies of KcsA K + channel appears to favour the classical snug-fit model [5] , [6] , a number of different mechanisms have been proposed to explain potassium channel selectivity, including the thermodynamic [7] , electrostatic [8] , [9] or geometric [10] differences in Na + and K + binding within the filter, to name a few. Our recent studies on NaK, a non-selective cation channel, and its mutants offer a wealth of direct insight into the structural details underlying tetrameric cation channel selectivity [11] , [12] ( Fig. 1 ). The NaK channel has a similar overall structure as KcsA with the exception that its selectivity filter has a sequence of 63 TVGDGN 68 , which forms two ion-binding sites, structurally identical to sites 3–4 of KcsA. Although K + ions bind within each site in a similar manner to K + -selective channels, NaK is completely non-selective and equally permeable to Na + and K + . On the basis of NaK, two sets of mutagenesis studies were performed. In the first set of mutants, collectively named NaK2CNG, the NaK filter was replaced with those commonly seen in eukaryotic cyclic nucleotide-gated (CNG) channels [13] . The selectivity filter of these NaK2CNG mutants have three in-line ion-binding sites equivalent to sites 2–4 of KcsA, yet the channels are still unable to discriminate between Na + and K + . In a separate set of mutations on the NaK channel, replacement of Asp66 and Asn68 to Tyr and Asp, respectively, convert NaK into a highly K + -selective channel, named NaK2K, with a filter containing four ion-binding sites superimposable with those of KcsA. These structural studies of NaK and its mutants demonstrate that irrespective of any other mechanisms involved, four contiguous ion-binding sites in the filter is a prerequisite for selective K + conduction. 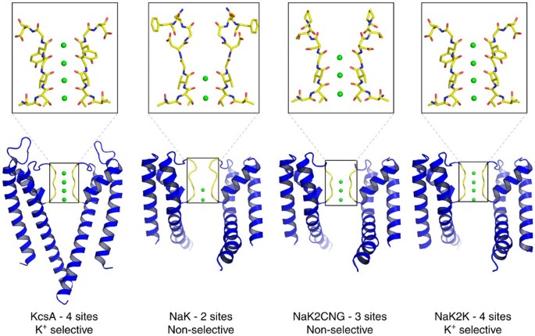Figure 1: Structure of K+selective and non-selective channels. The overall and filter structure (inset) of the K+selective KcsA and NaK2K channels, and the non-selective NaK and NaK2CNG channels. K+ions within the filter are represented as green spheres. Figure 1: Structure of K + selective and non-selective channels. The overall and filter structure (inset) of the K + selective KcsA and NaK2K channels, and the non-selective NaK and NaK2CNG channels. K + ions within the filter are represented as green spheres. Full size image As both NaK2K and NaK2CNG channels can be structurally determined to very high resolution and their selectivity measured directly by single-channel recording using giant liposome patch, these NaK mutants provide powerful tools for the precise examination of ion binding and selectivity within both K + -selective and non-selective channel filters. Here we probe how sodium–potassium competition alters K + occupancy at each site within the selectivity filter of NaK2K and NaK2CNG, and how this competition differs between selective and non-selective channels. Our results demonstrate that on competition of high Na + concentration, the K + -selective NaK2K maintains two high-affinity K + -binding sites (site 1 or 2) and prevent the permeation of Na + . Interestingly, although NaK2CNG still retains one high-affinity K + site (site 3) consistent with the thermodynamic affinity measurement using isothermal titration calorimetry (ITC) presented in the companion paper, the channel is still non-selective in Na + –K + permeation [14] . These observations demonstrate that although ion binding may be K + -selective to a single site, selective yet efficient conduction is a consequence of the multi-ion filter with multiple selective sites. Electrophysiology of K + and Na + competition in NaK2K Although highly selective for K + with the permeability ratio ( P Na / P K ) of 0.04 (ref. 13 ), NaK2K can also conduct Na + in the absence of K + without inactivation, albeit with much lower conductance ( Fig. 2a ). However, a low concentration of K + can block a large portion of the Na + current, whereas further increases in K + concentration lead to a significant increase in current, carried predominantly by K + ( Fig. 2a ). In the presence of about 150 mM Na + , the maximum blockage of the Na + current occurs at about 0.3 mM K + ( Fig. 2b ). This so-called anomalous mole fraction (AMF) effect of two permeable ions is also observed in MthK and other K + channels [15] , [16] , and is a key property of multi-ion pores [17] , [18] . As K + channel are classically described as being selective for K + primarily in comparison with Na + , the millimolar range concentration of extracellular K + under physiological condition would be sufficient to prevent Na + permeation. 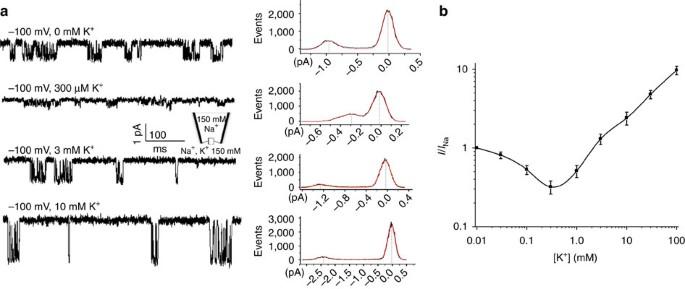Figure 2: Electrophysiology of Na+–K+competition in NaK2K. (a) Sample traces (left) and histograms (right) of single-channel currents at −100 mV through NaK2K at various concentrations of K+in bath solution. The pipette and bath solutions contain 150 mM Na+and 150 mM Na+–K+mixture, respectively. (b) Magnitude of the inward current (defined as the current from bath to pipette) as a function of potassium concentration. Data were normalized to the Na+current measured in the absence of K+(0 mM K+). Data points are mean±s.e.m. from five separate patches. Figure 2: Electrophysiology of Na + –K + competition in NaK2K. ( a ) Sample traces (left) and histograms (right) of single-channel currents at −100 mV through NaK2K at various concentrations of K + in bath solution. The pipette and bath solutions contain 150 mM Na + and 150 mM Na + –K + mixture, respectively. ( b ) Magnitude of the inward current (defined as the current from bath to pipette) as a function of potassium concentration. Data were normalized to the Na + current measured in the absence of K + (0 mM K + ). Data points are mean±s.e.m. from five separate patches. Full size image K + and Na + competition within the NaK2K filter To provide a structural perspective of how K + and Na + compete for the ion-binding sites in a K + -selective multi-ion pore, we performed a systematic crystallographic titration experiment in which crystals of the NaK2K channel, normally obtained in the presence of 150 mM KCl, were soaked in a series of stabilization solutions containing a NaCl–KCl mixture (150 mM total) at various ratios. The structures of these soaked crystals were determined and the ion occupancy at each site were analysed and compared. One technical challenge is the difficulty in differentiating the contributions of Na + , K + and, possibly, water molecules to the electron density in the selectivity filter even with high-resolution structures, making it almost impossible to determine ion occupancy simply based on the intensity of electron density. This difficulty can be partially overcome by calculating anomalous difference Fourier maps of soaked crystals. In our crystals, anomalous scattering is dominated by K + ions, whereas signals from Na + or oxygen (water) are negligible at the typical X-ray data collection wavelength of 1.0–1.5 Å ( Supplementary Table S1 ). Although weak, the high-resolution diffraction and minimal radiation damage to the crystals allow for sufficient quality data to measure this anomalous difference between Friedel pairs ( Supplementary Table S2 ). To enhance the anomalous signal, all data were collected at a wavelength of 1.5 Å, at which the anomalous scattering of K + is doubled as compared with that at 1 Å. This use of K + anomalous scattering effectively simplifies the assay by only measuring the K + occupancy change, which, combined with conventional analysis of electron density change, provides a quite accurate picture of K + –Na + competition at each site within the filter. 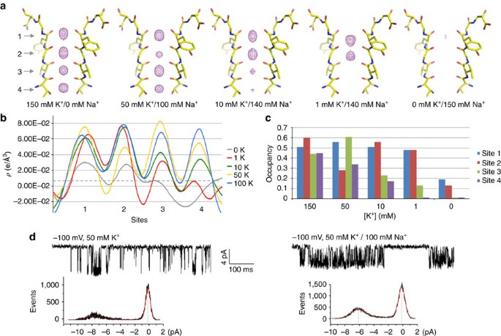Figure 3: Crystallographic titration of Na+–K+competition in NaK2K. (a) Anomalous difference Fourier maps (contoured at 0.03 e Å−3), (b) 1D anomalous difference density profiles along the central filter axis and (c) estimated occupancies of K+within the filter of NaK2K at various concentrations of K+. Dotted line indicates the baseline used for peak integration. (d) Single-channel traces and histograms of K+currents in NaK2K measured with 50 mM symmetrical KCl in the absence (left) and presence (right) of 100 mM Na+. Figure 3a shows the ensemble of the anomalous difference maps of the crystals titrated with various ratios of K + –Na + . The selectivity filter of NaK2K remained in a conductive conformation without observable structural change throughout the titration from high to low K + concentrations. All data used for map calculation were scaled with a common reference data (crystal with 150 mM K + in this case). At 150 mM K + , both the anomalous difference map and the conventional F o − F c ion omit map ( Figs 3 and 4 ) show four equivalent density peaks within the filter, indicating almost equal occupancy of K + ions at sites 1 through 4. On the basis of previous studies, on average, two K + ions are occupying the filter at high concentration and this would yield an occupancy of ~50% at each site [15] , [19] . At lower K + concentrations, although the contribution of Na + or water to the electron density in conventional F o − F c ion omit maps obscures K + binding within the filter, the anomalous difference maps provide a clear picture of the K + occupancy change at each site. This can be more quantitatively demonstrated in the one-dimensional (1D) profile of anomalous signal along the central axis of the filter ( Fig. 3b ). Assuming the four anomalous peaks at high K + reflect the anomalous scattering from two K + ions, we can also roughly estimate the K + occupancy at each site during titration by integrating the area under the peaks of the 1D anomalous electron density profile ( Fig. 3c ). Figure 3: Crystallographic titration of Na + –K + competition in NaK2K. ( a ) Anomalous difference Fourier maps (contoured at 0.03 e Å −3 ), ( b ) 1D anomalous difference density profiles along the central filter axis and ( c ) estimated occupancies of K + within the filter of NaK2K at various concentrations of K + . Dotted line indicates the baseline used for peak integration. ( d ) Single-channel traces and histograms of K + currents in NaK2K measured with 50 mM symmetrical KCl in the absence (left) and presence (right) of 100 mM Na + . 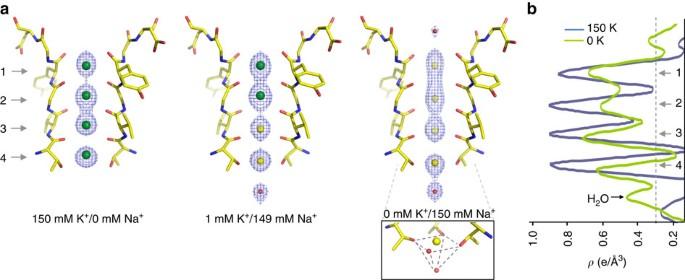Figure 4: Comparison of Na+and K+binding in NaK2K. (a)Fo−Fcion omit maps at the filter region of the NaK2K crystals soaked in 150 mM K+(left), 1 mM K+/149 mM Na+(centre) and 0 mM K+/150 mM Na+(right) contoured at 6σ. K+and Na+ions are drawn as green and yellow spheres, respectively. Inset depicts the coordination of the Na+bound at site 4 by the Thr63 hydroxyls and a water molecule in the cavity. (b) 1DFo−Fcelectron-density profiles along the central filter axis of NaK2K in 150 mM K+or 150 mM Na+(0 K). Full size image Figure 4: Comparison of Na + and K + binding in NaK2K. ( a ) F o − F c ion omit maps at the filter region of the NaK2K crystals soaked in 150 mM K + (left), 1 mM K + /149 mM Na + (centre) and 0 mM K + /150 mM Na + (right) contoured at 6 σ . K + and Na + ions are drawn as green and yellow spheres, respectively. Inset depicts the coordination of the Na + bound at site 4 by the Thr63 hydroxyls and a water molecule in the cavity. ( b ) 1D F o − F c electron-density profiles along the central filter axis of NaK2K in 150 mM K + or 150 mM Na + (0 K). Full size image One clear trend in the titration assay is that K + binding to the bottom two sites is diminishing at lower K + concentrations, as indicated by the disappearance of the K + anomalous signal, whereas the K + ions retain tight binding to the top two sites (sites 1 or 2). Even with only 1 mM KCl, the anomalous signals from the top two sites remain as intense as under high K + concentration, indicating equivalent occupancy. In light of the close proximity of these adjacent sites, this observation implies a single K + bound at low concentration, either at site 1 or 2. This preference of K + binding to the top two sites of the NaK2K filter is distinct from what was observed in MthK, where K + prefers sites 1 and 3 (ref. 15 ). This difference in site preference for K + ions between NaK2K and MthK is intriguing, as both channels have virtually identical filter structure. The cause of such difference is unclear and requires further investigation. With the removal of K + at the bottom two sites, the electron density at sites 3 and 4 observed in F o − F c ion omit map at low K + must be from Na + or water ( Fig. 4 ). Although difficult to distinguish, we believe that site 4 is mainly occupied by Na + based on its in-planar configuration with respect to the Thr63 hydroxyl oxygen ligands and the nearby water density in the cavity that is not observed in the K + -only crystals [11] ( Fig. 4a ). Another interesting observation in the crystals soaked with 50 mM K + /100 mM Na + is that the K + ions are unevenly distributed across the filter, with sites 1 and 3 having higher K + occupancy than sites 2 and 4 ( Fig. 3 ). The K + occupancy of site 1 and 3 is even higher than that under the 150 mM K + -only condition. This uneven distribution of K + is not observed in the crystals soaked in the 50 mM K + -only solution ( Fig. 5 ), indicating that the imbalanced K + binding is a result of Na + competition, probably at site 4. As a Na + ion is commonly seen at site 4 of NaK2K in low K + concentration ( Fig. 4 ), its competitive binding would destabilize K + ions bound in the 2, 4 configuration. The imbalanced K + occupancy between the 1,3 and 2,4 configurations would imply a less optimal K + permeation [20] . Indeed, in the presence of 100 mM Na + in addition to 50 mM K + , the channel exhibits a decrease in conductance in comparison with that measured with the 50 mM K + -only solution ( Fig. 3d ). 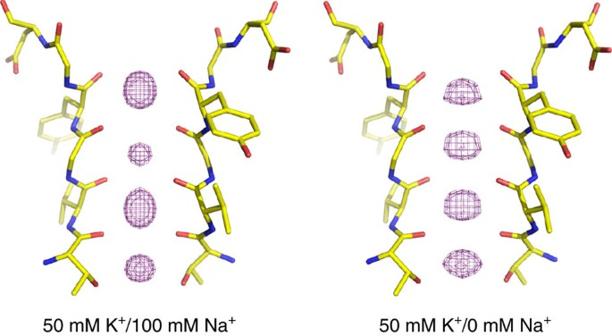Figure 5: Dependence of K+binding on competing Na+in NaK2K. Anomalous difference Fourier maps, contoured at 0.03 e Å−3, of K+bound within the NaK2K filter in the presence (left) and absence (right) of sodium. Figure 5: Dependence of K + binding on competing Na + in NaK2K. Anomalous difference Fourier maps, contoured at 0.03 e Å −3 , of K + bound within the NaK2K filter in the presence (left) and absence (right) of sodium. Full size image Na + binding in the K + -selective NaK2K filter As NaK2K is capable of conducting Na + in the absence of K + without undergoing inactivation, the soaking experiment also allows us to analyse how Na + binds within a conductive K + channel filter. Although trace amounts of K + still remain bound to the top two sites in crystals soaked in the Na + -only solution, as indicated by the weak K + anomalous signal, the electron density observed in the F o − F c ion omit map predominantly comes from Na + and water. As discussed, the Na + at site 4 tends to reside in plane with the hydroxyl oxygen ligands and a water molecule in the cavity participates in the pyramidal Na + coordination ( Fig. 4 ). Unlike discrete K + binding at the centre of each site, Na + binding to the top three sites is less well defined, as demonstrated by the broader distribution of electron density from the top edge of site 1 to the centre of site 3 ( Fig. 4 ). This diffusive density probably represents Na + residing in a continuum of states, from the centre of each ion-binding cage to the carbonyl oxygen plane. The density peaks at the centre of each binding site indicate that the centre position is slightly preferred for Na + binding. Electron density of water at the external entrance, not observed in the NaK2K–K + complex, probably participates in chelating the Na + at the top edge of site 1 in plane with the four carbonyl oxygen atoms from Tyr66. A similar Na + -binding scheme at site 1 is also observed in MthK [15] . The diffusive density with the NaK2K–Na + complex would suggest the lack of specific high-affinity Na + binding within the top three sites of the NaK2K filter. K + and Na + competition in the non-selective NaK2CNG channel The titration assay of the K + -selective NaK2K lead us to examine how K + and Na + compete in a non-selective filter. To test whether competition is a simple concentration-dependent linear displacement, we performed a similar titration assay using a non-selective NaK mutant, NaK2CNG_D, whose selectivity filter contains three contiguous sites superimposable with sites 2–4 of NaK2K. Maintaining 100 mM total salt concentration from the initial crystal condition, Fig. 6 shows the ensemble of the anomalous difference maps of the NaK2CNG_D crystals titrated with various mixtures of KCl–NaCl, as well as the anomalous signal 1D profile along the central axis of the filter. Similar to NaK2K, the NaK2CNG filter does not undergo observable structural change on ion exchange from high to low K + concentrations. At high K + , the three K + anomalous density peaks within the filter are equivalent, indicating equal K + occupancy. This would imply a population of 1.5 K + ions on average in the filter, probably representing an equal distribution between the configuration of two ions occupying sites 2 and 4, and the configuration of a single ion at site 3. To our surprise, despite it being non-selective in ion permeation, thermodynamically the NaK2CNG_D filter still prefers K + binding, particularly at site 3. As demonstrated in the 1D profile of the K + anomalous signal, although K + occupancy at sites 2 and 4 decrease with reduced K + concentration, the K + anomalous signal remains quite steady at site 3 even at 1 mM K + /99 mM Na + , indicating high-affinity K + binding ( Fig. 6b,c ). The apparent difference between NaK2K and NaK2CNG_D at low K + concentration is that NaK2K has two high-affinity sites (sites 1 and 2), whereas NaK2CNG has one at site 3. On removal of K + , the electron density within the top two sites (site 2 and 3) of NaK2CNG_D becomes diffusive, similar to what was observed in NaK2K, indicating the lack of specific Na + binding ( Fig. 7 ). The Na + ion at site 4 resides at the lower edge with a water molecule participating in the pyramidal coordination as commonly seen in all NaK mutants [11] , [21] . 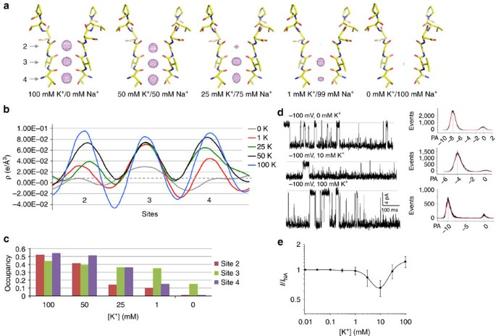Figure 6: Crystallographic titration of Na+–K+competition in NaK2CNG. (a) Anomalous difference Fourier maps (contoured at 0.03 e Å−3), (b) 1D anomalous difference density profiles and (c) estimated occupancies of K+within the NaK2CNG filter from crystals soaked in 100 mM Na+–K+mixture with various ratio. Dotted line indicates the baseline used for peak integration. (d) Sample traces and histograms of single-channel currents at −100 mV through NaK2CNG at various concentrations of K+. The pipette and bath solutions contain 150 mM Na+and 150 mM Na+–K+mixture, respectively. (e) Relative magnitude of the inward current with increasing potassium in bath solution. Data were normalized to the Na+current measured in the absence of K+ (0 mM K+). Data points are mean±s.e.m. from three separate patches. Figure 6: Crystallographic titration of Na + –K + competition in NaK2CNG. ( a ) Anomalous difference Fourier maps (contoured at 0.03 e Å −3 ), ( b ) 1D anomalous difference density profiles and ( c ) estimated occupancies of K + within the NaK2CNG filter from crystals soaked in 100 mM Na + –K + mixture with various ratio. Dotted line indicates the baseline used for peak integration. ( d ) Sample traces and histograms of single-channel currents at −100 mV through NaK2CNG at various concentrations of K + . The pipette and bath solutions contain 150 mM Na + and 150 mM Na + –K + mixture, respectively. ( e ) Relative magnitude of the inward current with increasing potassium in bath solution. Data were normalized to the Na + current measured in the absence of K+ (0 mM K + ). Data points are mean±s.e.m. from three separate patches. 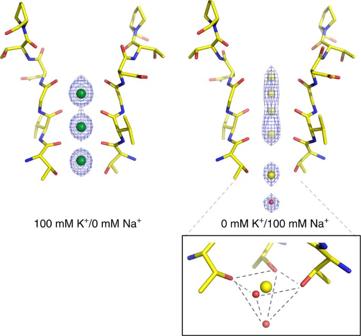Figure 7: K+and Na+binding in the filter of NaK2CNG. Fo−Fcion omit maps of the K+(left) and Na+(right) complexes of NaK2CNG contoured at 6σ. (Inset) Na+binding in plane with the Thr63 side-chain hydroxyls and a water molecule participate in the coordination from the bottom. K+and Na+ions are shown as green and yellow spheres, respectively. Full size image Figure 7: K + and Na + binding in the filter of NaK2CNG. F o − F c ion omit maps of the K + (left) and Na + (right) complexes of NaK2CNG contoured at 6 σ . (Inset) Na + binding in plane with the Thr63 side-chain hydroxyls and a water molecule participate in the coordination from the bottom. K + and Na + ions are shown as green and yellow spheres, respectively. Full size image The preference of K + in NaK2CNG_D can also be demonstrated in ion permeation measurements with a mixture of Na + and K + ( Fig. 6d,f ). The AMF effect of K + on Na + currents is observed in NaK2CNG_D but with two major differences as compared with NaK2K. First, the K + blockage of the Na + current is much weaker in NaK2CNG_D and occurs at about 10 mM. The second key difference is that the Na + current in NaK2CNG_D is much higher than that in NaK2K and comparable to the K + only current. Consistent with the weak AMF effect between Na + and K + in NaK2CNG, the selectivity measurement performed under mixed ions (135 mM K + /15 mM Na + in the pipette and 135 mM Na + /15 mM K + in the bath) instead of bi-ionic condition did show slight K + selectivity for NaK2CNG with reversal potential of about 15 mV ( P K / P Na ~2; Fig. 8 ). 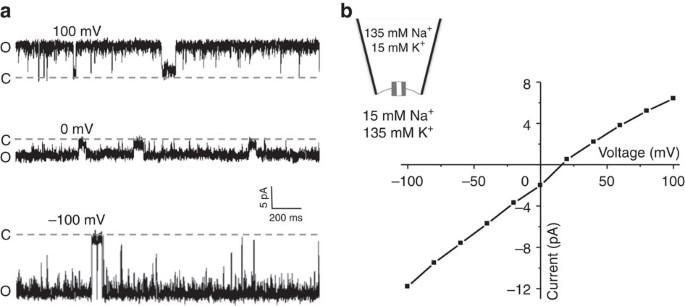Figure 8: Electrophysiology of ion selectivity in the NaK2CNG_D channel. Sample single-channel traces (left) andI–Vcurve (right) of NaK2CNG_D recorded using giant liposome patch clamping with 135 mM Na+/15 mM K+in the pipette and 15 mM Na+/135 mM K+in the bath. Figure 8: Electrophysiology of ion selectivity in the NaK2CNG_D channel. Sample single-channel traces (left) and I – V curve (right) of NaK2CNG_D recorded using giant liposome patch clamping with 135 mM Na + /15 mM K + in the pipette and 15 mM Na + /135 mM K + in the bath. Full size image A persistent, central question to understanding K + channels is the origin of K + selectivity. Our crystallographic titration experiments examine the structural basis of K + selectivity at thermodynamic equilibrium. Although the crystallographic titration may not provide an accurate measurement of the binding affinities of K + or Na + , by utilizing high-resolution structures along with anomalous signals, we can accurately define how Na + and K + compete in the K + -selective NaK2K and the non-selective NaK2CNG channels. The structural observation of concentration-dependent ion replacement within the filter, combined with single-channel electrophysiology, provides intriguing insights into the general mechanisms underlying selective ion permeation in K + channels. Under high Na + -low K + conditions, our titration assay reveals two adjacent high-affinity K + sites (sites 1 and 2) in NaK2K, allowing K + to effectively block the permeation of Na + . The presence of two high-affinity K + sites is also observed in MthK, although they are at sites 1 and 3 in that channel [15] . Despite this differnce, both channels share several key features in a high Na + –low K + environment. They both maintain two high-affinity K + sites occupied by a single K + ion of equal distribution between the two sites. In addition, site 1 appears to be a common K + -selective site in both channels and is likely to be also true for other K + channels as demonstrated in various electrophysiological studies on BK [22] , KcsA [23] and inward-rectifier K + channels [24] . Interestingly, the NaK2CNG channel (NaK2CNG_D in this study), whose ion permeation is non-selective under bi-ionic condition, still retains a highly K + -selective site at site 3 in its filter, as demonstrated in our crystallographic titration assay and the ITC titration (see companion paper) (ref. 14 ). With the presence of a single K + high-affinity site, K + can still somewhat block the permeation of Na + ( Fig. 6d,e ), but with a much weaker potency than that observed in NaK2K. One key difference between the affinity measurement by crystallographic or ITC titration and the reversal potential measurements for ion selectivity is that the former was performed under thermodynamic equilibrium, whereas the latter reflects a dynamic process of ion permeation across the filter. The lack of selectivity in NaK2CNG suggests that a single high-affinity K + site alone does not generate high K + selectivity during ion permeation. The ion-binding differences between NaK2K and NaK2CNG allows us to elucidate the interplay between thermodynamic binding and the dynamic process of ion conduction ( Fig. 9 ). Even with a high-affinity site at equilibrium, the apparent K + affinity during ion permeation is expected to be much lower due to the electrochemical driving force and the electrostatic repulsion of ions binding nearby. Assuming an apparent K d of 10 mM for the single K + -selective site in NaK2CNG, as inferred from the K + -blocking assay, that would give rise to a k off of about 10 7 s −1 ( K d = k off / k on with k on at the diffusion limit of 10 9 M −1 s −1 ), which is equivalent to pA current and, therefore, would not lead to significant blockage of a Na + current. In the presence of two K + -selective sites in a row, as seen in NaK2K, the K + -blocking effect will be significantly enhanced at low concentration. For simplicity, we assume both sites have the same apparent K d of 10 mM and a single K + ion has to move sequentially from one site to the other before exiting the pore. The k on of K + at the second site is determined by its k off from the first, which will have the limit of about 10 7 M −1 s −1 , and therefore the k off of K + at the second site would be <10 5 s −1 . This off rate after the second site is equivalent to a single ion blocking with higher apparent affinity of 0.1 mM, which is very close to the observed apparent K d (~0.3 mM) of the K + blocking of the Na + current in NaK2K. Thus, the presence of two K + high-affinity sites creates a double barrier for K + movement across the multi-ion filter at low concentration, and thereby effectively blocks the Na + current. It has been shown that the last K + ion in the Shaker K + channel filter leaves at a rate of about 10 5 s −1 (ref. 25 ), similar to what is calculated here. The principle of this double barrier to single K + permeation requires two K + -selective sites within the multi-ion pore but does not need to define the particular sites; as in NaK2K the high-affinity sites are 1 and 2, and in MthK they are sites 1 and 3. 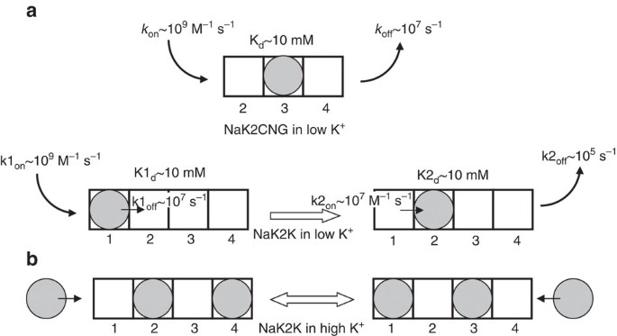Figure 9: Mechanism of K+blocking and permeation. (a) Mechanism of K+blocking of Na+currents in NaK2CNG and NaK2K at low potassium concentrations. (b) K+permeation through NaK2K at high concentration. Figure 9: Mechanism of K + blocking and permeation. ( a ) Mechanism of K + blocking of Na + currents in NaK2CNG and NaK2K at low potassium concentrations. ( b ) K + permeation through NaK2K at high concentration. Full size image In essence, K + -channel selectivity is defined by two processes: the blockage of Na + permeation at low K + concentration, which requires high-affinity K + binding, and a high flux rate at high K + concentration, which requires low-affinity binding. K + channel achieve these two seemingly mutually exclusive properties by having multiple (four) in-line ion-binding sites, two of which are highly K + selective. The above discussion describes the K + permeation and blockage with single occupancy at low concentration. At high K + concentration, the channel is converted from blocking mode to conducting mode by having two K + ions in the filter, hopping between two energetically equivalent configurations (1,3 and 2,4) (ref. 20 ). The entrance of a third K + at one end propels the exit of K + from the other end of the filter by mutual repulsion, analogous to Newton balls. Therefore, the double occupancy of K + in the filter effectively reduces the ion displacement mechanism from two steps, seen with single occupancy, to one step with double occupancy. Furthermore, the electrostatic repulsion of the two K + ions in the filter also reduces the K + affinity [26] , allowing for faster K + displacement. Protein expression and purification All proteins used for both structural and functional study were expressed and purified as previous described [13] , [27] . Briefly, the NaK double-mutant NaK2K, containing the mutations D66Y and N68D, or chimera NaK2CNG_D, where the filter sequence of 63 TVG DGNFS is replaced with with 63 TVG DTPP , were encoded in the pQE-60 vector and expressed in the Escherica coli strain SG13009. Expression was induced with 0.4 mM IPTG (isopropyl-β- D -thiogalactoside) in the presence of 5 mM BaCl 2 for 18 h at 25 °C. Cells were lysed in 100 mM KCl, 50 mM Tris–HCl, pH 8.0, solublized with 40 mM N -decyl-b- D -maltoside (DM) and purified on Talon IMAC column (Clontech). Eluted protein was digested overnight with thrombin, 1 unit thrombin per 2 mg protein, and further purified on a Superdex-200 (10/30) size exclusion column in 100 mM KCl, 20 mM Tris–HCl, pH 8.0, and 5 mM DM. An additional mutation, F92A, which increases flux through the channel, was generated using the Strategene Quick Change II mutagenesis kit for all channels used in functional studies. Crystallization Purified NaK2K and NaK2CNG_D channels were concentrated to ~20 mg ml −1 and crystallized in the same conditions previous described using sitting drop vapour diffusion at 20 °C. All crystals were initially grown in complex with K + by mixing equal volumes of protein solution with a well solution of 62.5–70% (±)MPD ((±)-2-methyl-2,4-pentanediol) and 100 mM buffer at various pH (2-( N -morpholino)ethanesulfonic acid for pH 6.5, HEPES for pH 7.0–7.5, Tris–HCl for pH 8.0–8.5). In all soaking experiments, the crystal was soaked overnight in stabilization solution containing 70% MPD, 10 mM DM, 100 mM Tris–HCl, pH 8.0 (for NaK2K), or 100 mM HEPES, pH 7.5 (for NaK2CNG_D), and defined mixtures of NaCl and KCl. The total salt concentration was maintained at 100 and 150 mM for NaK2CNG_D and NaK2K crystals, respectively. All crystals were flash frozen in liquid nitrogen, with stabilization solution serving as the cryoprotectant. All crystals were of the I 4 space group with unit cell dimensions around a = b =68 Å and c =89 Å, and contained two molecules in the asymmetric unit. The fourfold axis of channel tetramer coincided with the crystallographic tetrad. Data collection and structure determination X-ray diffraction data were collected at the Advanced Light Source beamlines 8.2.1 and 8.2.2, and the Advanced Photon Source 23-ID beamline. Data were processed and scaled in HKL2000 (ref. 28 ). Data were collected at 8,500 eV (~1.5 Å wavelength) to maximize the K + anomalous signal. Although all crystals diffracted to better than 2 Å ( Supplementary Table S2 ) due to the wavelength and limitations in the minimum detector distance at some beamlines, resolution at the edge of the detector was ~2.2 Å for some data. All data sets were therefore truncated to 2.2 Å for map calculation. As all crystals for soaking experiment were obtained from the same crystallization conditions as previously determined structures, the structures of NaK2CNG_D (PDB code 3K03) or NaK2K (PDB code 3OUF) were directly used in the refinement against the diffraction data of each soaking crystal in Phenix [29] , with solvent molecules and filter ions omitted. Model phases from partially refined structures were used for map calculation. All filter ions in figures were placed in COOT [30] using F o − F c ion omit maps. All NaK2K and NaK2CNG data were scaled against their respective potassium complex crystals before map calculation. F o − F c maps were calculated as omit maps with ions removed from within the filter. 1D electron-density profiles through the filter were calculated as previously described [20] by sampling the F o − F c and Fourier difference maps along the C axis using MAPMAN [31] . For occupancy estimation, the total area of the anomalous peaks above the baseline in 1D profile was set to represent two K + ions in the NaK2K–K + complex (total four peaks) and 1.5 ions in the NaK2CNG–K + complex (total three peaks); the area of individual peak at various [K + ] was then normalized against the total area to calculate the K + occupancy at each site. Electrophysiology For single-channel recordings, a protein/lipid (palmitoyloleoylphosphatidylethanolamine/palmitoyloleoylphosphatidylglycerol 3:1) ratio of 0.05–0.1 μg mg −1 was used to reconstitute proteoliposomes. Giant liposomes were obtained by air drying 2–3 μl of liposome sample on a clean cover slip overnight at 4 °C followed by rehydration in bath solution at room temperature. Patch pipettes were pulled from Borosilicate glass (Harvard Apparatus) to a resistance of 8–12 MΩ filled with pipette solution containing 150 mM NaCl, 1 mM EGTA, 10 mM HEPES, pH 7.4 buffered with NaOH. The bath solution contains 150 mM NaCl, 10 mM HEPES, 1 mM EGTA, pH 7.4, buffered with Tris. A gigaseal (>10 GΩ) was obtained by gentle suction when the patch pipette attached to the giant liposome. To get a single layer of membrane in the patch, the pipette was pulled away from the giant liposome and the tip was exposed to air for 1–2 s. Membrane voltage was controlled and current recorded using an Axopatch 200B amplifier with a Digidata 1322A digitizer (Axon Instruments). Currents were low-pass filtered at 1 kHz and sampled at 20 kHz, except the NaK2K patch with 300 μM KCl, which was filtered at 500 Hz due to the small currents. Only patches containing a single channel were used for further experiments. For the AMF measurement, NaCl in the bath solution was replaced by 150 mM mixture of NaCl–KCl, and the [K + ]-dependent single-channel current was recorded at −100 mV. The NaCl–KCl mixtures were prepared by mixing the solution of 150 mM NaCl, 1 mM EGTA, 10 mM HEPES, pH 7.4, buffered with NaOH and the solution of 150 mM KCl, 1 mM EGTA, 10 mM HEPES, pH 7.4, buffered with KOH at various ratios. Therefore, the only variable in these mixtures is the Na + /K + ratio. In each experiment of AMF measurements, the single-channel recordings at various K + concentrations were obtained from the same patch, with the recording time for each Na + /K + mixture longer than 3 min. The same experiments were repeated with five independent patches for NaK2K and three patches for NaK2CNG. All histograms of single-channel currents have bin-width of 0.01 pA, except the NaK2K patch with 300 μM KCl, which used a bin-width of 0.005 pA. Sodium block of potassium current was measured at −100 mV using 50 mM KCl and 10 mM HEPES buffered with KOH, pH 7.4, in both the pipette and bath solutions, in the presence or absence of an additional 100 mM NaCl added symmetrically, on both sides of the patch. Mixed ion selectivity of NaK2CNG_D was measured using solutions of 150 mM NaCl, 1 mM EGTA, 10 mM HEPES-NaOH, pH 7.4, and 150 mM KCl, 1 mM EGTA, 10 mM HEPES–KOH, pH 7.4, mixed at ratios of 9:1 in the pipette and 1:9 in the bath, respectively. All chemicals used for solution preparation were purchased from Sigma. How to cite this article: Sauer, D. B. et al. Sodium and potassium competition in potassium-selective and non-selective channels. Nat. Commun. 4:2721 doi: 10.1038/ncomms3721 (2013).